Human impacts drive a global topographic signature in tree cover The Anthropocene is a geological epoch marked by major human influences on processes in the atmosphere, biosphere, hydrosphere and geosphere. One of the most dramatic features of the Anthropocene is the massive alteration of the Earth’s vegetation, including forests. Here we investigate the role of topography in shaping human impacts on tree cover from local to global scales. We show that human impacts have resulted in a global tendency for tree cover to be constrained to sloped terrain and losses to be concentrated on flat terrain. This effect increases in strength with increasing human pressure and is most pronounced in countries with rapidly growing economies, limited human population stress and highly effective governments. These patterns likely reflect the relative inaccessibility of sloped topography and have important implications for conservation and modelling of future tree cover. Earth’s vegetation has undergone massives changes during the Anthropocene [1] , including the widespread conversion of forests to other land uses. Approximately 2.8 billion hectares of forest have been cleared for agriculture and harvest since 1850 (ref. 2 ), with profound consequences for atmospheric carbon pools [2] , [3] , [4] , biodiversity [5] and economic systems [6] . Clearing continues to threaten many remaining forests [7] , but land abandonment and afforestation are leading to forest expansion in other areas [8] , [9] . Conservation planning, prudent economic development and climate models [10] depend on accurate projections of tree cover under future land use and climate scenarios [11] , [12] . However, understanding the causes of deforestation has been challenging, in part because multiple ecological, political, economic and social factors can all be influential and interact over a vast range of spatial scales [13] . These difficulties are exacerbated by limited knowledge about the pattern and extent of deforestation [14] , [15] . We have some insight into the forces that influence tree cover dynamics at national scales [16] , [17] , [18] , and within local landscapes [19] , [20] , but little research has attempted to bridge this scale gap. Increases in the availability of remote-sensing data enable analyses of tree cover at a larger spatial extent and finer resolution than has previously been possible [7] . We take advantage of these developments to examine the role of climatic, anthropogenic and topographic drivers of tree cover across a wide range of scales. We particularly focus on topographic slope, because steep ground may act as a refuge for trees in human-dominated landscapes ( Fig. 1 ). This could be because sloped terrain is more difficult to clear, benefits obtained by clearing are lower [21] or the incentives to abandon cleared land are greater [22] . Topography has been shown to have important influences on tree cover at local or regional scales [19] , [20] , [23] , but the global generality of this remains untested. Indeed, many broad-scale studies of deforestation have focused primarily on economic factors, giving little attention to topographic and climatic effects [24] . 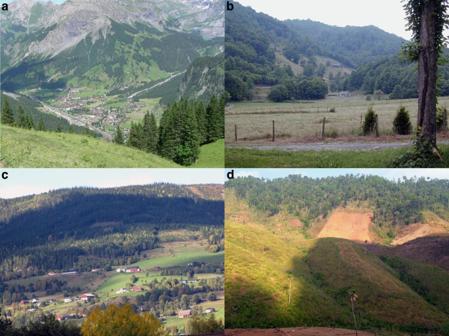Figure 1: Examples of anthropogenic associations between tree cover and topographic slopes. (a) Switzerland, 2008, (b) North Carolina, 2005, (c) Norway, 2012 and (d) Thailand, 2006. Clearing of trees for agriculture and housing tends to occur on relatively flat ground. Photos ina–cby J.-C.S. and indby Anders Barfod. Figure 1: Examples of anthropogenic associations between tree cover and topographic slopes. ( a ) Switzerland, 2008, ( b ) North Carolina, 2005, ( c ) Norway, 2012 and ( d ) Thailand, 2006. Clearing of trees for agriculture and housing tends to occur on relatively flat ground. Photos in a – c by J.-C.S. and in d by Anders Barfod. Full size image In this study, we use high-resolution (500 m), near-global (60°S to 60° N) estimates of per cent tree cover [25] derived from data from the satellite-borne Moderate Resolution Imaging Spectrometer (known as MODIS). We use these data to assess the impact of topography on tree cover across a wide range of spatial scales. Controlling for climatic variation, we then ask whether human land use drives the effects of topography. If human activities are at least partially responsible for the relationship between slope and tree cover, the social, political and economic context could modify this relationship [13] , [16] , [17] , [18] . For example, tropical deforestation rates have been shown to decrease as government becomes increasingly democratic [17] and the rule of law becomes more secure [16] . We address this possibility using a suite of country-level descriptors of the human context [26] and ask how these descriptors relate to the association between tree cover and slope. Further, MODIS tree cover estimates are made yearly, allowing us to also obtain an estimate of the rate of tree cover change through time. We use data obtained from 2000 to 2005. This provides a limited window to assess trends in tree cover; accordingly, we focus on describing the factors controlling tree cover change rather than on comprehensively assessing its magnitude. We find that both standing tree cover and tree cover increases are most pronounced on sloped terrain, whereas human impacts are strongest on flat terrain. In regions with very low human impacts, there is no association between tree cover and slope, strongly suggesting that this relationship is anthropogenic in origin. The strength of the relationship is affected by both climatic and socioeconomic factors, most notably population stress. Intensification of human land use in the coming century is likely to contribute to an increasingly strong limitation of the remaining tree cover to sloped terrain. Pattern of tree cover Tree cover and slope show a strong, general and global association ( Figs 2 and 3 ), suggesting that slopes indeed consistently act as refuges for trees. In contrast, human impacts are most pronounced on relatively flat terrain ( Supplementary Figs S1 and S2 ). The association of trees and slopes was particularly strong where human impacts are high ( Fig. 3c , Table 1 and Supplementary Fig. S3 ), supporting the hypothesis that the effect is anthropogenic in origin. Climate also modifies the strength of this effect; slopes are most important in regions with low-potential evapotranspiration (PET). 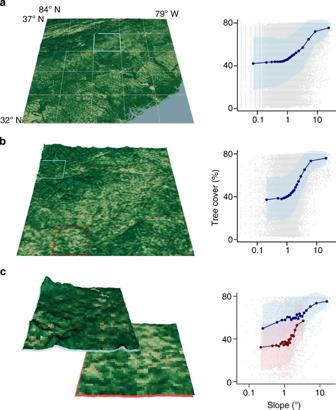Figure 2: Local examples of the relationship between topography and tree cover in the southeastern United States. The surface in each map represents elevation, and is coloured according to tree cover. (b,c) Zoomed-in views of particular regions withina, with moderate human impacts (b) and low (c, blue) or moderate impacts (c, red). The lines display tree cover means and s.d. for 20 slope quantiles. Figure 2: Local examples of the relationship between topography and tree cover in the southeastern United States. The surface in each map represents elevation, and is coloured according to tree cover. ( b , c ) Zoomed-in views of particular regions within a , with moderate human impacts ( b ) and low ( c , blue) or moderate impacts ( c , red). The lines display tree cover means and s.d. for 20 slope quantiles. 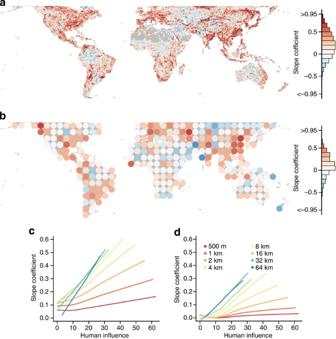Figure 3: Variation in the relationship between slope and tree cover. (a) A map of the relationship between topographic slope and tree cover, as estimated using standardized regression coefficients from models fit with 4-km cells within 120-km windows. Each window produced one coefficient estimate; the distribution of these local coefficients is shown in the histogram and is strongly skewed towards positive values. A similar relationship appeared at larger scales (32-km cells) for the relationship between tree cover change and slope (b). As mean human impacts within a window increased, the relationship between slope and tree cover (c) or tree cover change (d) within windows became stronger and more positive (as estimated using the slope coefficient from a multiple regression), especially at large spatial scales (lines display lowess regression fits). Full size image Figure 3: Variation in the relationship between slope and tree cover. ( a ) A map of the relationship between topographic slope and tree cover, as estimated using standardized regression coefficients from models fit with 4-km cells within 120-km windows. Each window produced one coefficient estimate; the distribution of these local coefficients is shown in the histogram and is strongly skewed towards positive values. A similar relationship appeared at larger scales (32-km cells) for the relationship between tree cover change and slope ( b ). As mean human impacts within a window increased, the relationship between slope and tree cover ( c ) or tree cover change ( d ) within windows became stronger and more positive (as estimated using the slope coefficient from a multiple regression), especially at large spatial scales (lines display lowess regression fits). Full size image Table 1 Predictors of local regression coefficients describing the importance of topographic slope for tree cover. Full size table The influence of slope on tree cover is scale-dependent ( Fig. 3c ). At small scales (500 m to 16 km), slope is a more important predictor than human impacts, precipitation or water deficit, and its importance increases with increasing scale up to grain sizes of 16 km ( Supplementary Fig. S4 ). However, at larger scales (16–512 km), the importance of slope declines and broad-scale climatic variation become substantially more important. This is consistent with strong small-scale variation in topography and human impacts, and the long-established importance of climate for the broad-scale distribution of vegetation [27] . It also suggests that coarse-grained studies, such as those using countries as the unit of analysis, are unlikely to detect a strong role for topography. Change in tree cover Between 2000 and 2005, there was a slight tendency towards gains in per cent tree cover. All continents held hotspots of tree loss, and all but Australia also had regions with substantial gains ( Supplementary Fig. S5 ). In contrast, forests (cells with >25% tree cover) tended to decline slightly between 2000 and 2005. These contrasting trends suggest a global reduction of forest cover that was offset by increasing densities of trees within remaining areas. This inference is consistent with recent increases of woody cover in savannahs, which may be attributable to atmospheric CO 2 increases [28] and with agricultural abandonment in regions such as eastern Europe, the former Soviet Union [9] and parts of Latin America [29] . In addition, focused afforestation programmes, notably in China, are leading to large increases in tree cover in some regions [8] . As expected under the hypothesis that slopes provide refuges for trees, decreases in cover were most probable on flat terrain ( Fig. 3b and Supplementary Fig. S6 ), particularly in areas with high human impacts ( Fig. 3d and Supplementary Fig. S7 ). This result was mirrored in a conservative analysis focused only on cells with both substantial tree cover (>25%) and cover change outside the range of uncertainty in the data (>15%), indicating that the effect of slope on tree cover change is robust ( Supplementary Figs S8 and S9 ). Although the importance of slope for the static pattern of tree cover peaked at intermediate scales, its importance for patterns of tree cover change increased monotonically with scale. Socioeconomic predictors Countries with large overall human impacts, strong environmental governance and limited population stress (low fertility rates and projected population growth) have the strongest relationships between slope and standing tree cover ( Fig. 4 and Supplementary Table S1 ). Slopes were most important as sites for expansion of tree cover between the years 2000 and 2005 in countries with limited population stress and low per-capita gross domestic product. Countries with low population stress were also most likely to experience increases in tree cover over this time period ( Supplementary Table S1 ). Overall, the association between tree cover and topography depends most strongly on the degree of population stress. This finding is consistent with expectations regarding forest regrowth after agricultural abandonment, which should be most common in sparsely populated areas [30] . Recent forest regrowth, for example, has been pronounced in Switzerland, a country with low population stress, high rates of agricultural abandonment and steep average slope [22] . These relationships may reflect the fact that both modern large-scale agriculture and increasing agricultural globalization facilitate geographic separation of production and consumption [29] . 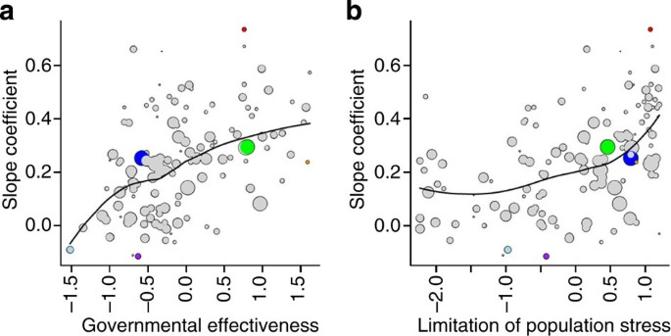Figure 4: The importance of slopes for tree cover. (a) Relationships between governmental effectiveness and slope and (b) the limitation of population stress and slope. Each point represents a country and is sized according to its area (log scale); lines display lowess regression fits. Six countries are highlighted: South Korea (red) had the strongest relationship between slope and tree cover, and the United States (green) and China (dark blue) are similar with respect to size and population stress, but quite different in governmental effectiveness. Denmark (orange) showed very high effectiveness and limited population stress but only moderately strong slope–tree cover relationships, perhaps because of its relatively flat topography. Iraq (light blue) and Syria (purple) had weak relationships between slope and tree cover. Figure 4: The importance of slopes for tree cover. ( a ) Relationships between governmental effectiveness and slope and ( b ) the limitation of population stress and slope. Each point represents a country and is sized according to its area (log scale); lines display lowess regression fits. Six countries are highlighted: South Korea (red) had the strongest relationship between slope and tree cover, and the United States (green) and China (dark blue) are similar with respect to size and population stress, but quite different in governmental effectiveness. Denmark (orange) showed very high effectiveness and limited population stress but only moderately strong slope–tree cover relationships, perhaps because of its relatively flat topography. Iraq (light blue) and Syria (purple) had weak relationships between slope and tree cover. Full size image These results provide a coherent global view of the factors controlling the distribution of forests across multiple spatial scales. Precipitation and water deficit appear to be primary drivers of the potential broad-scale distribution of trees ( Supplementary Fig. S4 ; together, these two variables explain 69% of variation in tree cover at the 128-km scale). Human impacts have reduced tree cover below this climatically defined potential, leading to the emergence of topographic slopes as important refuges for trees. This is particularly true in developed countries with low population growth rates, high economic growth and effective governments. The outstanding importance of population stress is consistent with the idea that increased pressure increases incentives to clear and utilize marginal land [18] . Anthropogenic deforestation ultimately reflects deliberate clearing of forests for agriculture, timber and construction, as well as unintentional declines in tree cover (for example, due to grazing). Forest regrowth, on the other hand, reflects socioeconomic dynamics such as the globalization of agriculture, politically determined re- and afforestation programmes and migration to urban areas and the associated land abandonment [8] , [9] , [29] . Our results show that these human impacts together drive a global topographic signature in tree cover. The association between topographic slope and tree cover was widespread ( Fig. 3a ) and detectable across a broad range of scales ( Fig. 3c ). This relationship was predicted based on previous small-scale research and expectations about the pattern of anthropogenic forest clearing. Nevertheless, human impacts may not provide the sole explanation for relationships between slope and tree cover. For example, the western slopes of the Sierra Nevada mountains in California receive more rainfall than the nearby Central Valley, which likely contributes to higher tree cover in the mountains. Such patterns are unlikely to explain our results in general, however, because climatic differences between adjacent mountains and plains are idiosyncratic and vary from region to region, we accounted for variation in climate in the regression models, and most important, across a wide range of scales, increasing human impacts led to stronger relationships between slope and tree cover, implicating human effects. Regions with minimal human impact showed almost no such relationship ( Fig. 3c ). As the human population increases and land use demands intensify over the next century of the Anthropocene, slopes are likely to become increasingly important refuges for forests. This has important implications for the future structure and function of forests. Complex topographies often provide heterogeneous habitat types, suggesting that sloped forests may harbour more biodiversity than nearby flat areas. Along elevational gradients, diversity is often highest at intermediate elevations, where slopes are likely to be most extreme and human impacts are often moderate. In this sense, the patterns of change in global tree cover are likely to produce smaller declines in biodiversity than would be expected under random loss. On the other hand, threatened species associated with lowland forests, such as the critically endangered lowland tree Glyptostrobus pensilis [31] , should be at greatest risk in the future. Limited data availability and incomplete integration of ecological and human-related causes have hampered understanding of the patterns and causes of deforestation. High-resolution remote-sensing data are collected repeatedly through time, objective and comparable among countries, promising to solve many data-related problems. The focus in discussions of forest cover dynamics has largely been on human aspects, but we show here that strong interactions between local topographic conditions and human impacts control tree cover distribution and dynamics. Predictive models of future changes in forest cover—with important impacts on livelihoods, biodiversity, water yield, the atmosphere and climate—need to take these interactions into account. Data sources Global estimates of tree cover were based on spectral data from the MODIS, using the vegetation continuous field algorithm. The data set is of high resolution, with a pixel size of 500 m, and contains an estimate of proportional tree cover for each pixel [7] , [25] . We used the distribution of trees in 2005 as our measure of the static pattern of tree cover. To estimate the per-year change rate for each cell, we fit a linear regression between year and tree cover for the cell in each year between 2000 and 2005. The slope of this regression was taken to be the tree cover change rate. In addition, we also produced conservative tree cover change maps that included cells that we were confident both had substantial tree cover (>25%) and had experienced a tree cover change outside of the MODIS vegetation continuous field range of uncertainty (a change of 15% in either direction). For the tree cover threshold, we considered any cell that had at least 25% tree cover in 2000 and that increased toward 2005, or any cell that had at least 25% tree cover in 2005, having declined from 2000. We explored a variety of potential climatic predictors of forest cover. In total, we considered eight potential predictor variables. These variables described total water availability (mean annual precipitation, MAP), energy availability (annual PET), water budget (annual water balance and total annual water deficit), seasonality of energy availability (temperature seasonality) and seasonality of water availability (precipitation seasonality, number of months with positive water balances and number of months with positive water balances and positive monthly mean temperature). All climate descriptors were obtained or derived from the WorldClim climate layers [32] , [33] . Topographic data were obtained from the Shuttle Radar Topography Mission. We used the 500-m CGIAR version 4 of the Shuttle Radar Topography Mission data, which have been processed to have data voids filled using other data sources and interpolation. We calculated topographic slope at the 500-m resolution, and aggregated this slope to lower resolutions as necessary. We used the Human Influence Index (HII), a unitless index that ranges from 0 (no impact) to 64 (maximum impact), to describe human land-use intensity [34] . HII combines information on population density, built-up areas, accessibility, landscape transformation and electric power infrastructure to estimate total human impacts within 30 arc-second grid cells globally. A major advantage of this index is that it is calculated in a globally consistent manner, ensuring comparability among regions. Scale A central goal of the analysis was to identify how changing spatial grain and extent affect the relationship between topographic variables, human land use, climate and tree cover. In part, this objective was inspired by the challenges inherent in the analysis of high-resolution global data sets. Such data allow detailed interpretation of relationships among variables over small spatial scales, but strong global trends can easily swamp these relationships. This may make it difficult to detect, for example, the effect of local slope on tree cover when it is incorporated into a global analysis that also includes major climatic drivers. We performed an analysis of the controls of tree cover at a series of nested scales. The spatial extents of analysis were 0.125, 0.25, 0.5, 1, 2, 4, 8, 16, 32 and 64° quadrats and global. For a given extent, we used rasters of each data layer at a resolution 1/30 the linear dimension of the extent. For example, for the smallest spatial extent of 1/8°, raw input data were 1/240° (the native resolution of the MODIS data, ~500 m at the equator) maps. We divided global maps of predictor and response variables of the appropriate resolution into a continuous grid of windows of the specified spatial extent and examined controls on tree cover within each of these windows. Climate model selection To select variables for use in the final regression models, we first considered collinearity among predictor variables. This model selection stage was conducted with data aggregated to a 1° resolution. We calculated variance inflation factors for each candidate predictor variable and removed strongly collinear variables until all variance inflation factor <10. Next, we assessed all possible linear combinations of the remaining predictor variables, and compared candidate models using the Bayesian information criterion. The best-performing model contained four predictor variables: MAP, annual PET, Deficit and precipitation seasonality. However, a simpler, two-variable model including only MAP and Deficit explained almost as much variation in tree cover. We retained these two models for all analyses, combining the climate predictors with slope and HII to obtain a ‘full model’ (six predictor variables) and a ‘reduced model’ (four predictor variables). The primary purpose of the climate portions of the models was to control for climatic effects on tree cover to allow clear detection of the effects of topography and human impacts. Of secondary interest was the interpretation of the parameter estimates of the climate variables themselves. Distributions of trees We calculated the total coverage of trees in 2000 and 2005 between 60° S and 60° N by multiplying the map of per cent tree cover at the full 500-m resolution by a map of cell area (accounting for latitudinal variation in cell size). We also applied a threshold of 25% to the tree cover rasters to obtain a binary map of forest distribution [7] . Analysis Within each window for a given spatial extent (and associated resolution), we determined the number of cells that had data values for all predictors. For any window that had at least 100 land cells (of the 900 possible cells) and for which tree cover varied within the window, we fit the full and reduced models. Forest cover and the HII were square-root-arcsine transformed, precipitation and precipitation seasonality were square-root transformed, and slope and deficit were log transformed. All variables were transformed to a s.d. of one and mean of zero to yield standardized regression coefficients. We also calculated the bivariate correlations between each predictor variable and tree cover. We analysed patterns of standardized regression coefficients and correlation coefficients among windows, across spatial scales and as a function of climate variables. Across all windows at a particular spatial scale, we calculated the median regression coefficient for each predictor variable for bivariate relationships, the full model and the reduced model, if appropriate. We then asked how these coefficients shift as a function of climate and spatial scale. We portrayed the relationships between a climate variable and a particular set of within-window coefficient estimates at a particular scale using lowess regression, a locally weighted regression technique. To describe these relationships statistically, we used ordinary least-squares and simultaneous autoregressive (SAR) models with local coefficient estimates from reduced models as the response variable and all environmental descriptors (calculated as mean values within each window) as the predictor variables. As computing SAR models for large data sets is computationally limiting, we subsetted the data to up to 2,000 randomly selected points for this analysis (for large spatial scales with <2,000 points, we used all available data). We fit error SAR models considering five different specifications of the neighbourhood weights matrix and selected the matrix that best removed spatial autocorrelation from model residuals (assessed using correlograms). The neighbourhood matrix was defined as all cell pairs less than 3,000 km apart, all cell pairs less than 1,000 km apart and all cell pairs less than x km apart, where x is the minimum distance that gives a neighbour for each cell, the nearest three neighbours of each cell and the nearest five neighbours of each cell. In all cases, the spatial weights matrix was row standardized [35] . In all but one case, the second definition removed the most spatial autocorrelation; the exception was tree cover change at the largest scale, for which we selected definition 4. Political and economic predictors We also performed analyses at the scale of nations to facilitate incorporating political and economic variables into the description of tree cover and tree cover change. For these analyses, we aggregated all above variables to the country level, and added information on per-capita gross domestic product, change in per-capita gross domestic product from 2000 to 2005 (ref. 36 ) and components of the Environmental Sustainability Score [26] . These component scores (and some of the areas they summarize) were in the following categories: Population Stress (incorporating fertility rates and projected population growth rates), Environmental Governance (incorporating various measures, including land protection, environmental knowledge and governmental effectiveness), Eco-efficiency (measures of energy efficiency and sustainability), Private Sector Responsiveness (various measures of the ‘greenness’ of business), Science and Technology (education rates, measures of innovation and percentage of population in research) and Participation in International Collaborative Efforts (international funding of environmental projects and participation in international agreements and organizations). We computed linear models predicting forest cover in 2005, forest cover change, or the mean coefficient relating slope and tree cover (at resolutions of 500 m, 4 km and 32 km) for each country based on all of the above predictor variables. To reduce this large model in each case, we calculated all possible subsets of it and selected the model with the lowest Akaike information criterion score. In all cases, regression models were weighted by the log(area) of each country. How to cite this article: Sandel, B. & Svenning, J.-C. Human impacts drive a global topographic signature in tree cover. Nat. Commun. 4:2474 doi: 10.1038/ncomms3474 (2013).